Solution-processed hybrid perovskite photodetectors with high detectivity Photodetectors capture optical signals with a wide range of incident photon flux density and convert them to electrical signals instantaneously. They have many important applications including imaging, optical communication, remote control, chemical/biological sensing and so on. Currently, GaN, Si and InGaAs photodetectors are used in commercially available products. Here we demonstrate a novel solution-processed photodetector based on an organic–inorganic hybrid perovskite material. Operating at room temperature, the photodetectors exhibit a large detectivity (the ability to detect weak signals) approaching 10 14 Jones, a linear dynamic range over 100 decibels (dB) and a fast photoresponse with 3-dB bandwidth up to 3 MHz. The performance is significantly better than most of the organic, quantum dot and hybrid photodetectors reported so far; and is comparable, or even better than, the traditional inorganic semiconductor-based photodetectors. Our results indicate that with proper device interface design, perovskite materials are promising candidates for low-cost, high-performance photodetectors. Photodetectors that capture light signals and convert them into electric signals are very important functional components in many applications [1] , [2] , [3] . A semiconductor material is essential to absorb the incident photons and create electron and hole pairs upon photo-excitation. And a built-in or applied electric field is necessary to separate the electrons and holes to produce an electric current. Various types of semiconductor materials have been applied in photodetectors, such as Si, InGaAs, ZnO, GaN, carbon nanotubes, quantum dots and conjugated polymers [1] , [2] , [3] , [4] , [5] , [6] , [7] , [8] , [9] , [10] . Although certain applications require different features, the key figure-of-merit parameters are responsivity ( R ), detectivity ( D *), noise equivalent power (NEP), linear dynamic range (LDR) and response speed. As briefly introduced later, we evaluate the photodetector performance on the basis of these parameters. Recently, a group of organic/inorganic hybrid perovskite materials were reported with rapid progress in photovoltaic cells [11] , [12] , [13] , [14] , [15] . Various device architectures have been demonstrated with respectable efficiencies of ~15% from simple solution processes [16] , [17] , [18] . More importantly, the long charge carrier lifetime and diffusion length have been observed from perovskite films showing low recombination of charge carriers in the bulk films. This strongly suggests a huge potential of this class of materials for solar cell and photodetector applications [19] , [20] , [21] , [22] . We observed perovskite materials with very high external quantum efficiency (EQE) in the spectral range from 300 to 800 nm, which is desirable for photodetector purposes. Also, it has been proposed that these types of materials have a very low density of defects and traps within the bandgap [23] . It suggests that the saturation current ( J 0 ) of the perovskite-based diodes can be very low. The absorption coefficient ( ε ) of the hybrid perovskite reaches the order of 10 4 cm −1 , which can be ascribed to the direct bandgap nature of the electronic transition. Therefore, a very thin (few hundred nanometres) layer of the material is sufficient for almost complete light absorption. With such a thin film, the travel distance for photogenerated charge carriers is small, and thus the photoresponse should be fast. These characteristics strongly indicate that the hybrid perovskite materials are ideal candidates for photodetector applications. Given the above-mentioned advantages of the material’s properties, we demonstrate a novel solution-processed hybrid perovskite photodetector. By using a water/alcohol-soluble conjugated polymer as the hole-blocking layer, we reduced the dark current density and achieved a very high detectivity for the hybrid perovskite photodetectors. In addition, our devices work at low (or even zero) bias, and show large dynamic linear response range, fast response speed as well as low noise currents. The parameters are compatible or even better than those of the commercial Si photodetectors. Our results indicate that the hybrid perovskite material is a promising candidate for low-cost and high-performance photodetectors. Organic–inorganic hybrid perovskite photodetector design The device structure of our photodetector is shown in Fig. 1a and the energy diagram of the device is shown in Fig. 1b . On top of indium tin oxide (ITO)-coated glass, an organic–inorganic hybrid CH 3 NH 3 PbI 3− x Cl x layer was sandwiched between PEDOT:PSS (hole-transporting material, p-type layer) and PCBM (electron-transporting material, n-type layer). Solar cells based on similar configuration have been demonstrated with fairly good performance in previous reports [24] . To reduce the charge recombination as well as the dark current density under reverse bias (particularly important for photodetectors), 2,9-dimethyl-4,7-diphenyl-1,10-phenanthroline (BCP) and poly[(9,9-bis(3′-( N , N -dimethylamino)propyl)-2,7-fluorene)-alt-2,7-(9,9-dioctylfluorene)] (PFN) were used as the contact buffer materials. Aluminium was used as the top electrode. Three types of devices were fabricated: PD1 without buffer, and PD2 and PD3 with BCP and PFN as cathode buffer layers, respectively. 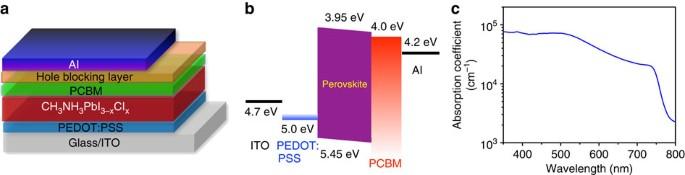Figure 1: Hybrid perovskite photodetectors. (a) Device structure of the hybrid perovskite photodetector. (b) Energy diagram of the perovskite photodetector under a slight reverse bias. (c) UV–visible absorption spectra of the photodetector without the hole-blocking layer and the Al electrode. Figure 1c shows the absorption spectrum of the photodetector (buffer layer and Al electrode are not included). The absorption onsite is at 780 nm and the device has a strong absorption from the near-IR to UV region, which mainly comes from CH 3 NH 3 PbI 3− x Cl x (absorption coefficient over 10 4 cm −1 ). The thickness of the active layer was varied from 200 to 600 nm, and it was found that a thickness over 300 nm is enough to absorb most of the photons (see Supplementary Fig. 1 for the absorption profiles at different film thicknesses). Figure 1: Hybrid perovskite photodetectors. ( a ) Device structure of the hybrid perovskite photodetector. ( b ) Energy diagram of the perovskite photodetector under a slight reverse bias. ( c ) UV–visible absorption spectra of the photodetector without the hole-blocking layer and the Al electrode. Full size image Detectivity characterization Responsivity, the ratio of photocurrent to incident light intensity, indicates how efficiently the detector responds to an optical signal. It is expressed as, where J ph is the photocurrent and L light is the incident light intensity. Since R is proportional to the quantum yield of the photodetector, it is very important for a photodetector to have a high conversion rate from photons to electrons/holes, or high EQE. Detectivity is given by where A is the effective area of the detector, f is the electrical bandwidth and i n is the noise current. When the dark current is dominated by the shot noise, D * can be expressed as where J d is the dark current and q is the elementary charge. Evidently, the dark current of the diode should be depressed as low as possible to distinguish from very weak optical signals. To obtain a small J d , the semiconductor film should have low trap density, low thermal emission (recombination) rates and good film quality to avoid any leakage current during operation. To characterize the photodetector, we used a light-emitting diode working in continuous mode as a monochromatic light source. 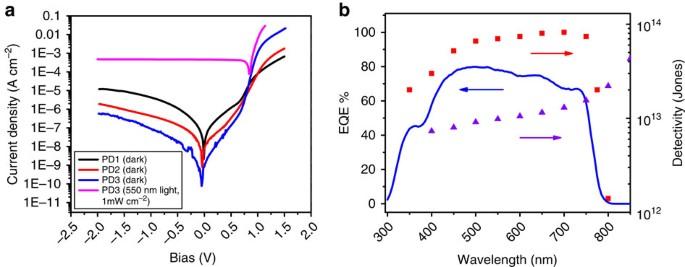Figure 2: Performance of hybrid perovskite photodetectors. (a) Current density–voltage curves of photodetectors with and without the hole-blocking layer. PD1, without hole-blocking layers; PD2, with BCP as the hole-blocking layer; and PD3, with PFN as the hole-blocking layer. (b) External quantum efficiency and detectivity of the hybrid perovskite photodetector at different wavelength. The detectivity of a single-crystalline silicon diode (purple triangle) is shown for comparison. Figure 2a shows the current density–voltage ( J – V ) characteristics measured in the dark and under illumination with λ =550 nm (power density=1 mW cm −2 ). All devices show similar photocurrent densities under light (see Supplementary Fig. 2 for the J – V curves). Because the photocurrents remain almost constant at different reverse bias (0 to −2 V), a very small (or even zero) voltage can be applied to extract the electrons and holes generated in the detector. The dark J – V characteristics, however, vary markedly. For PD1, a rectification ratio of ~10 2 (±1 V) and a dark current density of 1 × 10 −7 A cm −2 (at −100 mV) were obtained. The specific detectivity at 550 nm was then calculated to be 3 × 10 11 Jones (Jones=cm Hz 1/2 W −1 ). The large J d indicates significant injection under reverse bias. One possible reason is that the contact between the PCBM layer and the Al cathode causes hole injection into the diode. To verify whether hole injection occurs in PD1, a layer of BCP, which is famous for its hole-blocking properties due to its deep HOMO level of −6.7 eV (ref. 25 ), was deposited on PCBM. As expected, PD2 showed a smaller J d and a higher detectivity of 2 × 10 12 Jones at −100 mV. Interestingly, when PFN was used, PD3 showed a significantly reduced J d , a good rectification ratio of ~10 5 (±1 V) and a very high detectivity of 8 × 10 13 Jones at −100 mV. Note, the hybrid perovskite photodetectors can also be self-powered and work at 0 bias. If calculated at 0 mV, the detectivity is as high as 4 × 10 14 Jones ( J d at 0 mV is lower and getting close to the noise current). PFN has been widely used in organic light-emitting diode and organic photovoltaic devices because it builds up the surface dipole to lower the work function of metal cathode, and improves the electron injection and extraction in those devices [26] , respectively. Here it is found that PFN serves as an excellent hole-blocking material for photodetectors. The mechanism is believed to be similar to the organic light-emitting diode and organic photovoltaic devices. A dipole layer is formed at the PCBM and Al interface, which provides an extra electric field to prevent the hole injection while enhancing electron injection. This explains the marked increase in forward bias injection of PD3 in comparison with PD1 and PD2 as shown in Fig. 2a . The EQE and detectivity of the photodetector (PD3) at different wavelengths is shown in Fig. 2b . The device has a photoresponse from 300 to 800 nm and a peak EQE of 80%. From 350 to 750 nm, the detectivity approaches 10 14 Jones (at −100 mV), which is about one order of magnitude higher than the detectivity of a Si photodetector in the same spectral region (the detectivity of a Si photodetector is shown in Fig. 2b for comparison) [9] . Figure 2: Performance of hybrid perovskite photodetectors. ( a ) Current density–voltage curves of photodetectors with and without the hole-blocking layer. PD1, without hole-blocking layers; PD2, with BCP as the hole-blocking layer; and PD3, with PFN as the hole-blocking layer. ( b ) External quantum efficiency and detectivity of the hybrid perovskite photodetector at different wavelength. The detectivity of a single-crystalline silicon diode (purple triangle) is shown for comparison. Full size image The high detectivity of perovskite photodetectors is mainly due to its extremely low dark current under reverse bias. Interface engineering ensures a good blocking layer to avoid the leakage current; however, the dark current is ultimately limited by the recombination current, which is an intrinsic property of the semiconductor material and the heterojunction diode. To further understand this issue, we fit the dark J – V curve to extract the dark saturation current density, J 0 , a parameter that is directly related to the band-to-band thermal emission and recombination rate in semiconductors. As shown in Fig. 3 , our perovskite detector (PD3) has a very low J 0 of 1.5 × 10 −11 mA cm −2 (see Methods for detailed calculations), which is much lower than some of the conventional solution-processed semiconductor diodes such as CdTe (8 × 10 −11 mA cm −2 ) and GIGS (6 × 10 −7 mA cm −2 ) (ref. 27 ). Such a small J 0 explains the origin of its high photo-detectivity and also illuminates the reason why very small bandgap-to- V OC losses (~0.4 eV) can be achieved with perovskite-based photovoltaics [28] . 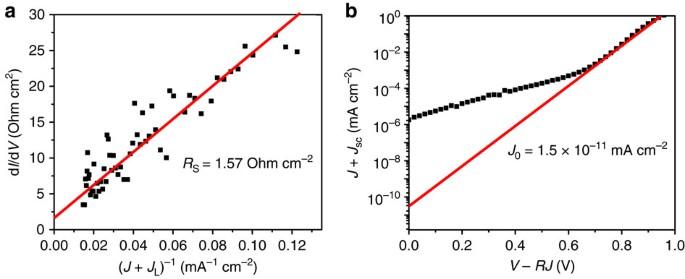Figure 3: Current–voltage characteristic the photodetectors (PD3). The device structure is ITO/PEDOT:PSS/CH3NH3PbI3−xClx/PCBM/PFN/Al. The originalJ–Vcurve is shown inFig. 1c. (a) Plot of −dV/dJvs (J+JL)−1and linear fitting. (b) ln(J+JSC) vs (V−RJ) and linear fitting. Both the fittings are located around the correspondingVOC. TheJ0is calculated to be 1.5 × 10−11mA cm−2. Figure 3: Current–voltage characteristic the photodetectors (PD3). The device structure is ITO/PEDOT:PSS/CH 3 NH 3 PbI 3− x Cl x /PCBM/PFN/Al. The original J – V curve is shown in Fig. 1c . ( a ) Plot of −d V /d J vs ( J + J L ) −1 and linear fitting. ( b ) ln( J + J SC ) vs ( V − RJ ) and linear fitting. Both the fittings are located around the corresponding V OC . The J 0 is calculated to be 1.5 × 10 −11 mA cm −2 . Full size image Another figure-of-merit for photodetectors is the LDR, or photo-sensitivity linearity (typically quoted in dB). Linear dynamic range is given by where is the photocurrent, measured at a light intensity of 1 mW cm −2 . It indicates that within a certain range, the photocurrent has a linear response as the incident light intensity changes. This is important because beyond this range the intensity of the light signal cannot be detected and calculated precisely. 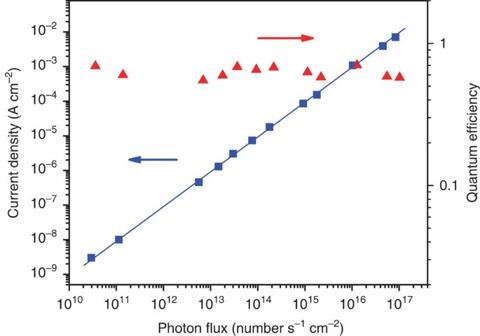Figure 4: Linear dynamic range of the photodetectors (PD3). The device structure is ITO/PEDOT:PSS/CH3NH3PbI3–xClx/PCBM/PFN/Al. The photodetector has a large linear dynamic range of >100 dB. Figure 4 shows photocurrent vs light intensity for PD3. When illuminated under light, the device shows a linear response within the incident photon flux density range from 10 17 to 10 10 number s −1 cm −2 (or power density range from 1 × 10 −1 to 1 × 10 −8 W cm −2 ) and a linear dynamic range of over 100 dB. These results are comparable with Si photodetectors (120 dB) and higher than other types of photodetectors such as InGaAs (66 dB). The quantum efficiency remains almost constant at different incident power density ( Fig. 4 , y axis on the right). Thus, we confirm that the hybrid perovskite photodetector is well suited to detect a wide range of incident powers. Figure 4: Linear dynamic range of the photodetectors (PD3). The device structure is ITO/PEDOT:PSS/CH 3 NH 3 PbI 3– x Cl x /PCBM/PFN/Al. The photodetector has a large linear dynamic range of >100 dB. Full size image Transient photocurrent response characterization The response speed of a photodetector is strongly related to charge transport and collection. Some devices need optical signals to be collected to enable operation with a certain bandwidth (for example, high-frequency optical communication), which requires fast extraction of photogenerated charge carriers. The transient time of free carriers can be controlled by the thickness of the active layer, applied electrical bias and the choice of interfacial charge transport materials. The response speed is another important parameter for photodetectors. The measurement of our hybrid perovskite photodetector (PD3) was performed under a 550-nm pulse light from a light-emitting diode. The rising and decay of the input pulse signal are within a few nanoseconds as calibrated by a single-crystalline Si photodiode ( Fig. 5a ). Devices with various film thicknesses were examined. As shown in Supplementary Fig. 3 , when the film thickness is ≪ 300 nm, there is no significant difference for the response speed. However, when the film is too thick (for example, 600 nm), the device shows much lower speed, most likely due to the increase of the charge carrier path length. To achieve sufficient light absorption, small leakage current and fast response simultaneously, devices with a thickness of ~300 nm are found to be optimal. Devices with an active area of 0.1 and 0.01 cm 2 were measured. 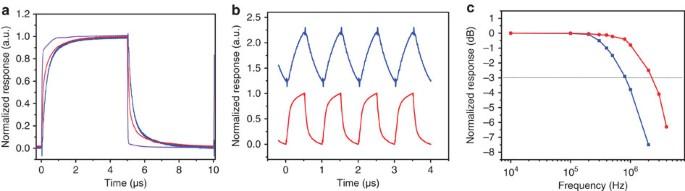Figure 5: Transient photocurrent response of the photodetectors with different device areas. (a) Transient photocurrent response at a pulse frequency of 100 kHz with a device area of 0.1 cm2(blue line) and 0.01 cm2(red line). Transient photocurrent response of a silicon diode is shown for comparison. (b) Transient photocurrent response at a pulse frequency of 1 MHz with a device area of 0.1 cm2(blue line) and 0.01 cm2(red line). (c) Frequency response of the photodetectors with a device area of 0.1 cm2(blue line) and 0.01 cm2(red line). Figure 5a shows the transient photocurrents of the devices measured under 0 bias at a light intensity of ~10 μW cm −2 and at a pulse frequency of 100 kHz (photoresponse of the silicon diode is shown for comparison). The transient response results for the device with 0.01 cm 2 area shows a rise time (output signal changing from 0 to 70% of the peak output value) of 180 ns and a decay time of 160 ns. The rise time and decay time for a device with 0.1 cm 2 area are both ~600 ns. Figure 5b shows the transient photocurrents at a pulse frequency of 1 MHz. Clearly, the small area device has rapid response rates and reaches ~80% of its maximum, whereas the response of the large area device is relatively slow. Figure 5c shows the normalized response vs pulse frequency for the devices. The 3-dB bandwidth decreased from 2.9 to 0.8 MHz when the device area increased from 0.01 to 0.1 cm 2 , because the speed is related to the RC constant of the circuit. It is noted that the response speeds of our perovskite photodetectors presented here are faster than most of the organic, quantum dot and hybrid photodetectors (typically on the order of millisecond) [4] , [5] , [6] , [7] , [8] , [9] , [10] and slightly slower than the silicon diode in Fig. 5a (≤20 ns). The speed is probably limited by the lower charge carrier mobility of the organic layer (PCBM, mobility ~10 −3 cm 2 V −1 s −1 ) (ref. 29 ) and the RC constant of the circuit [7] . When integrated into a circuit for real world applications, the pixel size should be much smaller and therefore the response speed of the perovskite photodetectors is predicted to be much faster. Figure 5: Transient photocurrent response of the photodetectors with different device areas. ( a ) Transient photocurrent response at a pulse frequency of 100 kHz with a device area of 0.1 cm 2 (blue line) and 0.01 cm 2 (red line). Transient photocurrent response of a silicon diode is shown for comparison. ( b ) Transient photocurrent response at a pulse frequency of 1 MHz with a device area of 0.1 cm 2 (blue line) and 0.01 cm 2 (red line). ( c ) Frequency response of the photodetectors with a device area of 0.1 cm 2 (blue line) and 0.01 cm 2 (red line). Full size image Noise current and noise equivalent power Noise equivalent power is another important figure-of-merit for photodetectors. It represents the minimum impinging optical power that a detector can distinguish from the noise. It is equal to the reciprocal of D * and can be expressed as To calculate NEP values for the hybrid perovskite photodetector (PD3), noise current of the devices were measured using a lock-in amplifier. The noise spectra at various frequencies are presented in Fig. 6a and the noise current plots at different dark current levels are shown in Fig. 6b . The noise current decreases at a higher frequency and increases at a larger reverse bias due to the larger dark current. The device shows small noise currents of ≪ 1 pA Hz −1/2 , which is about one order of magnitude smaller than that of a silicon diode [30] . The NEP of the photodetector is calculated to be 4.6 × 10 −12 W at 550 nm (−100 mV, 3 kHz) and 4.2 × 10 −12 W at 700 nm (−100 mV, 3 kHz). Very small noise currents at low bias are key for achieving such small NEP values for the hybrid perovskite photodetectors. 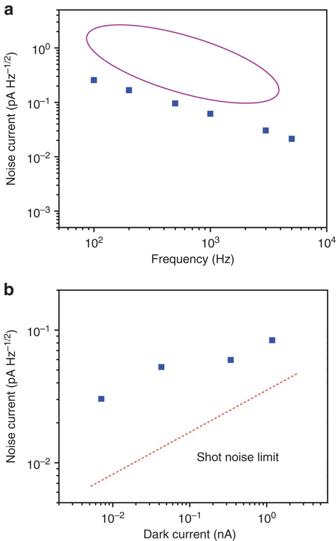Figure 6: Noise current of the photodetectors. (a) Measured dark current noise at different frequencies. The purple circle indicates reported values for a silicon photodiode. (b) Measured dark current noise at different dark currents. The shot noise limit is also plotted for comparison. Figure 6: Noise current of the photodetectors. ( a ) Measured dark current noise at different frequencies. The purple circle indicates reported values for a silicon photodiode. ( b ) Measured dark current noise at different dark currents. The shot noise limit is also plotted for comparison. Full size image The above results suggest the importance of designing device structure and selecting suitable interface materials for high photodetector performance. To explore the effects of device architecture on the photodetector performance, we also fabricated devices with a ‘regular’ structure: ITO/TiO 2 /CH 3 NH 3 PbI 3− x Cl x /p-doped spiro-MeOTAD/Au (PD4) (ref. 31 ). The photovoltaic performance was found to be similar to the device reported here (~14% power conversion efficiency). However, we noticed that the response speed for such device is rather slow ( Supplementary Fig. 4 ). In the transient photocurrent measurements, the device showed a response time of ~30 ms, which is 10 5 times longer than that of the inverted device using PEDOT:PSS and PCBM as the interface materials. Such a low speed is probably due to the slow response of the interface materials, particularly the lithium salt-doped spiro-MeOTAD [31] . Moreover, it was observed that when working in the photovoltaic mode, our inverted device showed a weaker hysteresis effect in the forward bias region compared with the regular device [31] (see Supplementary Fig. 5 for more details). The transient photocurrent response speed and the hysteresis effect may correlate with each other, suggesting that interface engineering is important for achieving high-speed photoresponse in photodetectors and minimizing hysteresis in photovoltaic cells. So far, the hysteresis effect in the perovskite photovoltaics is still under debate, and according to our results and other literature reports; the interface contact and the charge transport layers are probably the key issues. In summary, we have demonstrated the solution-processed high-performance photodetectors based on organic–inorganic hybrid CH 3 NH 3 PbI 3− x Cl x using an ‘inverted’ device configuration. The performance parameters of these photodetectors are comparable to or even better than photodetectors fabricated from vacuum-processed inorganic materials. Such high performance can be attributed to the excellent intrinsic optical and electronic properties of the hybrid perovskite as well as the judicious interface design. We believe that the hybrid perovskite materials can be used in a variety of low-cost photodetector applications and our results should inspire new fundamental studies on the properties of such materials. Materials PbCl 2 was purchased from Alfa Aesar. [6,6]-Phenyl-C 61 -butyric acid methyl ester (PCBM) was purchased from Nano-C. PEODT:PSS solution was purchased from Clevios. Unless otherwise stated, all of the chemicals were purchased from Aldrich and used as received. Device fabrication The device architecture of the photodetector is shown in Fig. 1a . The pre-cleaned ITO substrates were treated with UV ozone. A thin layer (~30 nm) of PEDOT:PSS (Baytron P VP A1 4083) was spin-coated onto the ITO surface that was pretreated by UV ozone for 15 min. After being baked at 150 °C for ~10 min, the substrates were transferred into a nitrogen-filled glovebox ( ≪ 0.1 p.p.m. O 2 and H 2 O). For the perovskite layer, PbCl 2 and CH 3 NH 3 I were dissolved in DMF in a 1:3 ratio. Specifically, the concentration of the PbCl 2 and CH 3 NH 3 I were 0.8 and 2.4 M. The solution was spin-coated onto the PEDOT:PSS layer at 800~2,000 r.p.m. (film thickness of 200~600 nm) and then annealed in air at 100 °C (on a hot plate) for 1 h. Subsequently, the devices were transferred into a glovebox and 2% PCBM in chlorobenzene solution was coated onto the perovskite layer at 1,000 r.p.m. For PD1, the film was then transferred into a thermal evaporator that is located in the same glovebox. For PD2, a thin layer of BCP (~5 nm) was coated on the PCBM layer by thermal evaporation. For PD3, a thin layer of PFN (~5 nm) was coated on the PCBM layer by spin coating. The device fabrication was completed by thermal evaporation of 100 nm Al as the anode under vacuum at a base pressure of 2 × 10 −6 torr. The effective area of film was measured to be around 0.10 or 0.010 cm 2 depending on the shadow mask that was used. Current–voltage characterization The fabricated devices were encapsulated in a nitrogen-filled glovebox by UV epoxy and cover glass. The current density–voltage curves were measured using an Agilent 4155C Semiconductor Parameter Analyzer. The devices were illuminated by monochromatic light from a light-emitting diode (550 or 700 nm). The light intensity was controlled by varying the voltage on the light-emitting diode. The actual light intensity was measured using a power meter. External quantum efficiencies were measured by an Enli tech (Taiwan) EQE measurement system. Dark JV curve analysis On the basis of the solar cell equivalent circuit, the J – V characteristics are described by: where J is the current flow through the external load, J SC is the light-induced current (for the dark J – V fitting, J SC =0). J 0 is the dark saturate current density, V is the applied voltage, A is the ideality factor, K B is the Boltzmann constant, T is the temperature and e is the electron charge. Equation 6 can also be written as and . The J 0 can be obtained by fitting the curve of ln( J SC − J ) vs ( V + R s J ), where the R s is obtained by fitting the curve of d V /d J vs ( J SC + J ) −1 . The plot of d V /d J vs ( J SC + J ) −1 and ln( J SC + J ) vs ( V − R s J ) are shown in Fig. 2 . From linear fitting of Fig. 2 , the device exhibited series resistance (~1. 57 Ω cm 2 ). By linear fitting the ln( J SC + J ) vs ( V − R s J ) ( Fig. 2 ), J 0 is calculated as 1.5 × 10 −11 mA cm −2 . Transient photocurrent measurements A light-emitting diode (550 nm) was modulated by the function generator as the excitation source. Square waves with different frequencies were applied. The photodetectors were directly connected to the oscilloscope (Tektronix DPO 4104) with an input impedance of 50 Ω. Noise current measurements Noise current was directly measured with a lock-in amplifier SR830. The photodetectors were kept in the dark room and shielded in Al foils during measurements. How to cite this article : Dou, L. et al. Solution-processed hybrid perovskite photodetectors with high detectivity. Nat. Commun. 5:5404 doi: 10.1038/ncomms6404 (2014).